An auto-inducible mechanism for ionic liquid resistance in microbial biofuel production Ionic liquids (ILs) are emerging as superior solvents for numerous industrial applications, including the pretreatment of biomass for the microbial production of biofuels. However, some of the most effective ILs used to solubilize cellulose inhibit microbial growth, decreasing efficiency in the overall process. Here we identify an IL-resistance mechanism consisting of two adjacent genes from Enterobacter lignolyticus , a rain forest soil bacterium that is tolerant to an imidazolium-based IL. These genes retain their full functionality when transferred to an Escherichia coli biofuel host, with IL resistance established by an inner membrane transporter, regulated by an IL-inducible repressor. Expression of the transporter is dynamically adjusted in direct response to IL, enabling growth and biofuel production at levels of IL that are toxic to native strains. This natural auto-regulatory system provides the basis for engineering IL-tolerant microbes, which should accelerate progress towards effective conversion of lignocellulosic biomass to fuels and renewable chemicals. Lignocellulosic biomass is an abundant resource that is available for the sustainable production of biofuels and high-value chemicals. Some of the most promising approaches have centered on engineering microbes [1] , [2] , [3] and utilizing a wide range of feedstocks, including woody biomass, indigenous grasses and agricultural residues such as corn stover [4] , [5] . The inherent recalcitrance of biomass requires an initial pretreatment step to render polysaccharides free from lignin for subsequent enzymatic or chemical hydrolysis to fermentable sugars. To solubilize lignocellulosic biomass, certain hydrophilic ILs are highly effective and environmentally friendly pretreatment agents that generate relatively low amounts of biomass-derived inhibitors compared with other conventional pretreatment methods [6] , [7] , [8] , [9] . A major disadvantage of the commonly used imidazolium ILs is their intrinsic microbial toxicity, which impairs growth of typical biofuel-producing hosts such as Escherichia coli and Saccharomyces cerevisiae , hence preventing efficient biofuel production [10] , [11] , [12] . In addition, the inhibition of biofuel synthetic enzymes by these ILs can severely reduce the yield of the final product [11] . It was recently demonstrated that an engineered E. coli strain is able to convert IL-pretreated biomass into biofuels in laboratory-scale experiments [5] . However, the extensive washing required for complete IL removal is not feasible in large-scale, industrial applications. An ideal and more sustainable process should balance the costs of removing IL with fermentation performance [13] . A novel way to achieve this would use biofuel-producing microbes that can tolerate residual levels (for example, 0.2–5% wt/vol) of ILs. Because a mechanism for microbial tolerance to ILs has not been elucidated, we investigated an IL-tolerant bacterium isolated from rain forest soils. Enterobacter lignolyticus grows well in at least 380 mM (5.5%) 1-ethyl-3-methylimidazolium chloride (abbreviated as [C 2 mim]Cl) [14] , [15] , an IL that is a promising pretreatment solvent for biomass [6] . Using RNA-sequencing transcriptomics, we determined that E. lignolyticus responds to [C 2 mim]Cl exposure by the differential expression of 688 genes, resulting in a complex response with numerous phenotypic changes [15] . These include an increased production of cyclopropane fatty acids, scavenging of compatible solutes and regulation of membrane transporters. Here we use a targeted functional screening approach, as a complement to the global nature of transcriptomics, to identify the key genetic elements responsible for [C 2 mim]Cl tolerance and discover that these consist solely of an efflux pump and its regulator. We transfer these genes to an engineered E. coli host, and demonstrate enhanced production of a terpene-based biofuel in the presence of this IL. A single gene is responsible for IL tolerance To cover a potentially complex IL-tolerance mechanism with many genes involved, we used relatively large DNA fragments (30–50 kb) to construct a fosmid library for screening in E. coli . Out of ~6,000 clones, 41 (0.7%) evinced an IL-tolerance phenotype by growing rapidly in the presence of 136 mM [C 2 mim]Cl. Sequence analysis of these clones revealed a common region of 2.6 kb encompassing three genes, only one of which was entirely represented ( Fig. 1a ). E. coli carrying this common region grew at rates similar to or greater than those of the source bacterium E. lignolyticus in a medium containing up to 410 mM [C 2 mim]Cl ( Fig. 1b ; Supplementary Fig. 1 ). This protective effect was not due to catabolism of the IL, as there was no measurable decrease in the [C 2 mim] + cation concentration after culturing cells to the stationary phase compared with the beginning of culture ( Supplementary Fig. 2 ). 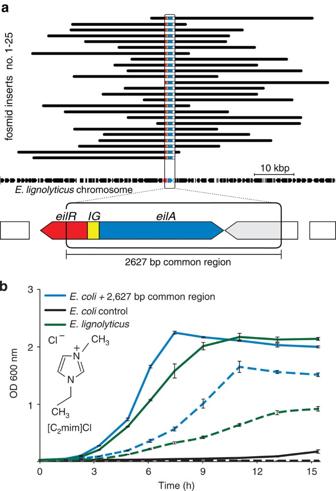Figure 1: Identification ofeilAby its function inE. coli. (a) AnE. colifosmid library containing fragments of genomic DNA fromE. lignolyticuswas screened for growth on [C2mim]Cl by plating cells directly following phage infection. After end-sequencing from the fosmid insertion sites of 25 [C2mim]Cl-tolerant clones, these sequences (black bars) were aligned with the genome ofE. lignolyticus. All inserts shared 2,627-bp (boxed region) containing the completeeilA(blue bar) and an adjacent section of theeilRregulatory gene (red bar). TheeilARmodule comprises these two genes and the 117-bp intergenic region (IG; yellow bar). (b) Growth ofE. lignolyticus(green curves), andE. colicontaining a plasmid, either without (black) or with the common region (blue) in 272 mM (solid line) and 410 mM (dashed line) [C2mim]Cl. The chemical structure of [C2mim]Cl is shown within the graph. The curves and error bars represent the means and standard deviation of biological triplicate measurements. Figure 1: Identification of eilA by its function in E. coli . ( a ) An E. coli fosmid library containing fragments of genomic DNA from E. lignolyticus was screened for growth on [C 2 mim]Cl by plating cells directly following phage infection. After end-sequencing from the fosmid insertion sites of 25 [C 2 mim]Cl-tolerant clones, these sequences (black bars) were aligned with the genome of E. lignolyticus . All inserts shared 2,627-bp (boxed region) containing the complete eilA (blue bar) and an adjacent section of the eilR regulatory gene (red bar). The eilAR module comprises these two genes and the 117-bp intergenic region ( IG ; yellow bar). ( b ) Growth of E. lignolyticus (green curves), and E. coli containing a plasmid, either without (black) or with the common region (blue) in 272 mM (solid line) and 410 mM (dashed line) [C 2 mim]Cl. The chemical structure of [C 2 mim]Cl is shown within the graph. The curves and error bars represent the means and standard deviation of biological triplicate measurements. Full size image The complete gene, designated eilA (Enterobacter IL tolerant; locus tag Entcl_2352), encodes a 52-kDa protein that is homologous to the ubiquitous major facilitator superfamily (MFS) of membrane transporters, although no orthologue is present in E. coli . The identification of this gene corroborates our previous observation that it is one of the most highly upregulated transcripts in E. lignolyticus when exposed to [C 2 mim]Cl [15] . Sequence analysis indicated that EilA is a homologue of proton antiporters, possessing 14 transmembrane helices that span the inner membrane. Numerous representatives of this MFS subgroup are responsible for prokaryotic and eukaryotic multidrug resistance, capable of transporting a range of hydrophobic cations, including some widely used bactericidal quaternary ammonium compounds and dyes [16] , [17] , [18] . Assuming a similar function of EilA, we screened a library consisting of 240 compounds representing many different structures and properties and found that EilA exports primarily hydrophobic ammonium cations ( Supplementary Data 1 ; Supplementary Fig. 3 ). It is noteworthy that E. coli expressing eilA is relatively resistant to methyl viologen (paraquat), a divalent bipyridinium cation. This observation is consistent with a group of efflux pumps that share up to 77% sequence identity to EilA, and which export methyl viologen from other Enterobacteriaceae, such as Salmonella and Klebsiella species [19] , [20] . We also examined the tolerance of an E. coli eilA strain to other imidazolium-based ILs, comparing different alkyl chain lengths at the N1 position on [C 2 mim] + and also replacing the Cl − anion with acetate. In general terms, we observed a correlation between an increase in alkyl chain lengths and toxicity, and that acetate was tolerated but to a lesser extent than Cl − ( Supplementary Figs 1 and 4 ). Expression is regulated by a [C 2 mim]Cl-inducible repressor In nature, bacteria are exposed to fluctuating concentrations of a broad spectrum of organic compounds. To respond to potentially toxic effects, expression of the appropriate transporters is typically adjusted by substrate-inducible transcriptional regulators [21] . The E. lignolyticus eilR gene (locus tag Entcl_2353), located upstream of eilA and only partially present on the 2.6-kb region, encodes a 22-kDa protein of the TetR family of transcriptional repressors ( Fig. 1a ). Proteins of this family are known to be prominent regulators of bacterial multidrug efflux pumps, including MFS transporters [22] . The 117-bp noncoding intergenic region ( IG ; Fig. 1a ) contains the predicted promoter and operator sequences for the two divergently transcribed genes. In experiments with E. coli that included only the IG - eilA sequence, [C 2 mim]Cl tolerance was maintained, confirming that the eilA promoter sequence resides within IG and is operational in E. coli ( Supplementary Fig. 5 ). To analyse the regulation of eilA expression, we measured the fluorescence of an EilA–green fluorescent protein (GFP) fusion protein, which confirmed that expression from the native promoter is constitutive. Introducing eilR into the cassette resulted in repression in the absence of [C 2 mim]Cl, whereas increasing the [C 2 mim]Cl level directly correlated with EilA–GFP expression ( Fig. 2a,b ). Therefore, we postulate that [C 2 mim]Cl induces the release of EilR from its operator site, resulting in activation of eilA transcription. A similar mechanism has been demonstrated by several studies on homologous Tet repressor-regulated efflux pump systems [22] , including the methyl viologen operon pqrAB in Streptomyces [23] . In the presence of 0.1 mM methyl viologen, E. coli expressing eilA constitutively grew at a near-normal rate. However, insertion of eilR in its native alignment (as eilAR ) resulted in complete growth inhibition. Moreover, when E. lignolyticus was exposed to methyl viologen, the lag phase was considerably prolonged ( Supplementary Fig. 6 ), indicating that EilR is not induced by this EilA substrate. Thus, in other phenotypic screening approaches, candidate genes such as those encoding efflux pumps could be overlooked when expression is restricted by substrate-specific transcriptional regulation. 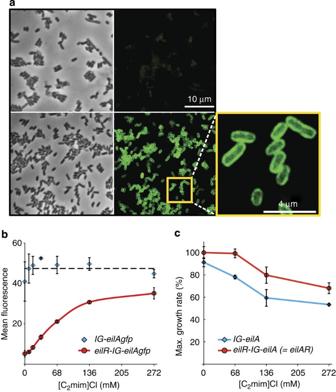Figure 2: [C2mim]Cl-inducible repressor EilR regulateseilAexpression. (a) Phase contrast (left) paired with fluorescence (right) microscopy images ofE. colicells expressing an EilA–GFP fusion protein from a plasmid carrying theeilR–IG–eilAgfpcassette. Cultures were grown in the absence of [C2mim]Cl (upper) or in the presence of 272 mM [C2mim]Cl (lower). The magnification shows membrane localization of EilA–GFP. (b) Mean single-cell fluorescence ofE. coliexpressing EilA–GFP from the native promoter, either constitutively (IG–eilAgfp: blue diamonds) or under the control of EilR (eilR–IG–eilAgfp: red circles). Cells were grown in the indicated [C2mim]Cl concentrations before flow cytometry measurements. The dashed line indicates the general trend. (c) Maximum growth rates ofE. coliexpressingeilAvia the native promoter, either constitutively (blue diamonds) or under the control of EilR (red circles). For bothbandc, the curves and error bars represent the means and standard deviation of biological triplicate measurements. Figure 2: [C 2 mim]Cl-inducible repressor EilR regulates eilA expression. ( a ) Phase contrast (left) paired with fluorescence (right) microscopy images of E. coli cells expressing an EilA–GFP fusion protein from a plasmid carrying the eilR–IG–eilAgfp cassette. Cultures were grown in the absence of [C 2 mim]Cl (upper) or in the presence of 272 mM [C 2 mim]Cl (lower). The magnification shows membrane localization of EilA–GFP. ( b ) Mean single-cell fluorescence of E. coli expressing EilA–GFP from the native promoter, either constitutively ( IG–eilAgfp : blue diamonds) or under the control of EilR ( eilR–IG–eilAgfp : red circles). Cells were grown in the indicated [C 2 mim]Cl concentrations before flow cytometry measurements. The dashed line indicates the general trend. ( c ) Maximum growth rates of E. coli expressing eilA via the native promoter, either constitutively (blue diamonds) or under the control of EilR (red circles). For both b and c , the curves and error bars represent the means and standard deviation of biological triplicate measurements. Full size image Overexpression of a transporter can overload the cell membrane and have deleterious consequences on cell viability [24] , which we observed when eilA was expressed at higher levels from an isopropyl-β- D -thiogalactoside-inducible promoter ( Supplementary Fig. 7 ). To prevent this while maintaining maximum export capacity of the inhibitory compound, a substrate-responsive efflux system has been suggested for biotechnological applications such as those used in biofuel production [25] . We confirmed this by testing the growth of E. coli strains over a range of [C 2 mim]Cl levels. Compared with a strain in which eilA is expressed constitutively under the control of its native promoter, higher growth rates were observed in the presence of the repressor ( Fig. 2c ). We reasoned that EilR increases cell viability by adjusting efflux pump expression to [C 2 mim]Cl concentration, so we included the entire native eilAR cassette in experiments using a biofuel-producing E. coli strain. Engineering an IL-tolerant biofuel production strain Bisabolane is an advanced biofuel candidate with combustion properties comparable to diesel. The dehydrogenated precursor, bisabolene, is produced from acetyl-coenzyme A (CoA) in E. coli with a two-plasmid system: one plasmid contains eight heterologous mevalonate pathway genes, and the other has the plant-derived bisabolene synthase gene [26] . We assembled these genes onto a single plasmid optimized for bisabolene production, then introduced a second plasmid containing the eilAR cassette to create a prototype IL-tolerant biofuel production system. To represent different possible fermentation scenarios, we tested cell growth and bisabolene production by this engineered E. coli strain in a medium containing a range of [C 2 mim]Cl concentrations from 0 to 270 mM, representing the residual [C 2 mim]Cl remaining with the hydrolysate after pretreatment and saccharification [13] . For E. coli lacking eilAR , increasing the [C 2 mim]Cl concentration in the growth medium caused a marked increase in lag time, up to 445% at 136 mM, and no growth was observed at 272 mM ( Fig. 3a ; Supplementary Fig. 1 ). Even at 63 mM [C 2 mim]Cl, the lowest level tested, a doubling in lag time would hamper the overall efficiency of a biofuel production process [3] . In contrast to the control, we found the growth of cultures expressing eilAR only slowed moderately with increasing [C 2 mim]Cl, to a maximum lag time increase of 120% at 272 mM. 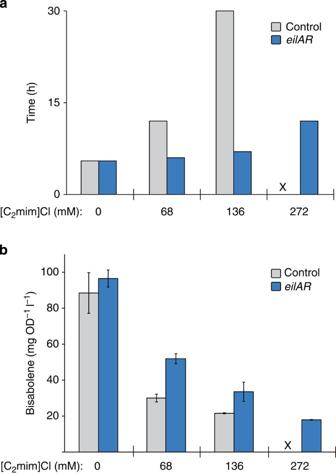Figure 3: Bacterial bisabolene production in media containing [C2mim]Cl. E. coliharbouring a plasmid containing the bisabolene pathway and a second plasmid either with theeilARcassette (blue bars) or lacking an insert as control (grey bars). (a) Time required for each culture to reach OD600nm=1, the standard cell density used for inducing the bisabolene pathway. (b) Bisabolene production measured 6 days after induction of cultures grown in three [C2mim]Cl concentrations, as indicated with columns and error bars representing the means and standard deviation of technical triplicate measurements. Values were normalized to cell density to illustrate productivity of the bacteria. X indicates that no growth or production was observed. Figure 3: Bacterial bisabolene production in media containing [C 2 mim]Cl. E. coli harbouring a plasmid containing the bisabolene pathway and a second plasmid either with the eilAR cassette (blue bars) or lacking an insert as control (grey bars). ( a ) Time required for each culture to reach OD 600nm =1, the standard cell density used for inducing the bisabolene pathway. ( b ) Bisabolene production measured 6 days after induction of cultures grown in three [C 2 mim]Cl concentrations, as indicated with columns and error bars representing the means and standard deviation of technical triplicate measurements. Values were normalized to cell density to illustrate productivity of the bacteria. X indicates that no growth or production was observed. Full size image Cultures were grown to the same cell density before inducing the biosynthetic pathway. Bisabolene production of both the eilAR and the control strain was similar in [C 2 mim]Cl-free medium, whereas the eilAR cassette enabled increased productivity over the control in the presence of [C 2 mim]Cl. In 68 mM [C 2 mim]Cl, cells expressing eilAR produced 52 mg OD 600 −1 l −1 bisabolene, 73% more than the control strain. This effect was apparent with increasing IL concentrations ( Fig. 3b , Supplementary Fig. 8 ). We observed decreased bisabolene production for both strains in [C 2 mim]Cl compared with the IL-free medium. Productivity decreased by 66% in the control and 46% in the eilAR strain in 68 mM [C 2 mim]Cl. Certain ILs have been shown to interfere with production of biofuels at levels below the growth inhibition threshold, most likely owing to direct inhibition of biosynthetic pathway enzymes. For example, bacterial biodiesel yield decreased by 25% in the presence of only 6 mM of an imidazolium-based IL [11] . In summary, we have shown that targeted, functional screening of DNA from environmental microorganisms is a powerful approach to discover the mechanisms underpinning phenotypes such as bacterial resistance to inhibitory compounds. Such mechanisms can include regulatory proteins that specifically respond to natural and synthetic inducer molecules. The sequence-independent method used here can be expanded to detect further mechanisms useful for engineering other IL-sensitive host organisms such as Clostridium spp. or Saccharomyces cerevisiae . In our case, transferring a genetic module from a rain forest soil microbe to an E. coli biofuel host conferred the tolerance needed for it to grow well in the presence of toxic concentrations of ILs. We demonstrated that this introduced efflux mechanism improved production of a biofuel precursor in the presence of low (residual) levels of an IL used in biorefineries ( Fig. 4 ). We anticipate that engineering IL-tolerant biofuel pathway enzymes and production strains with tolerance to inhibitors originating from biomass breakdown [27] are needed to further increase yields. Autoregulation of IL-efflux by the EilR repressor increased strain robustness and is particularly important for efficient production in industrial-scale fermentations, where residual IL levels fluctuate between biomass batches. In addition, such a substrate-responsive system obviates the need for costly inducer molecules. An IL-tolerant biofuel host could also convert the adverse effects of these solvents into an advantage by preventing growth of microbial contaminants, thus allowing fermentation under more economical, aseptic conditions. By eliminating a bottleneck of a promising biomass pretreatment method, our findings could contribute to an effective and sustainable production of biofuels and chemicals. 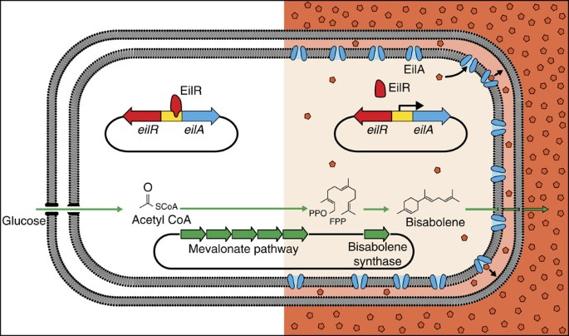Figure 4: Model of the ionic liquid-tolerant bacterium converting hydrolysed biomass into biofuel. The cell harbours a plasmid containing the bisabolene biosynthetic genes (green), and another plasmid with theeilARcassette encoding the efflux pump EilA (blue) and repressor EilR (red). Sugars from the hydrolysate are metabolized to acetyl-CoA, which then feeds into the biofuel production pathway (green arrows). In the absence of ionic liquid (left half), EilR binds to the operator in the IG (yellow), therefore preventingeilAtranscription. The presence of the cellulose solubilizing ionic liquid [C2mim]Cl (orange pentagons; right half) causes EilR to release from the operator site, resulting in EilA expression and membrane insertion. EilA then exports toxic [C2mim]Cl from the cell, enabling robust growth and efficient production of biofuels. Figure 4: Model of the ionic liquid-tolerant bacterium converting hydrolysed biomass into biofuel. The cell harbours a plasmid containing the bisabolene biosynthetic genes (green), and another plasmid with the eilAR cassette encoding the efflux pump EilA (blue) and repressor EilR (red). Sugars from the hydrolysate are metabolized to acetyl-CoA, which then feeds into the biofuel production pathway (green arrows). In the absence of ionic liquid (left half), EilR binds to the operator in the IG (yellow), therefore preventing eilA transcription. The presence of the cellulose solubilizing ionic liquid [C 2 mim]Cl (orange pentagons; right half) causes EilR to release from the operator site, resulting in EilA expression and membrane insertion. EilA then exports toxic [C 2 mim]Cl from the cell, enabling robust growth and efficient production of biofuels. Full size image Reagents All chemicals were purchased from Sigma-Aldrich. Fosmid library construction and screening To obtain genomic DNA, E. lignolyticus was cultivated in 10 ml Luria Bertani medium for 16 h at 30 °C, then centrifuged and cells resuspended in TE buffer to an OD 600 of 1. Lysozyme (1.7 mg ml −1 final concentration) was added to the cell suspension and incubated for 30 min at 37 °C. Following this, a standard cetyltrimethylammonium bromide method was used to extract genomic DNA [28] . The genomic DNA library was constructed in the pCC1FOS fosmid vector (Epicentre biotechnologies), using the manufacturer’s protocol, but the size separation step was omitted as the extracted DNA had the average size needed for fosmid cloning (~40 kb). A control library was built using 42-kb human control DNA. The titre of phage particles was determined for both E. lignolyticus and control libraries and diluted to receive ~1,500 clones per 120 mm × 120 mm plate. Infected E. coli EPI300 cells were spread directly on Luria Bertani agar plates containing 12.5 mg l −1 chloramphenicol and 136 mM [C 2 mim]Cl and incubated at 37 °C. After 20 h, the clearly detectable tolerant clones were selected from all four plates and grown overnight in media containing 0.01% arabinose to induce a high fosmid copy number. Fosmids were isolated using standard column DNA purification (Qiagen). The insert ends were sequenced using the suggested primers pCC1FOS-F (5′-GGATGTGCTGCAAGGCGATTAAGTTGG-3′) and pCC1FOS-R (5′-CTCGTATGTTGTGTGGAATTGTGAGC-3′). The sequences (600–1,000 bp) were then aligned to the E. lignolyticus genome (GenBank ID: CP002272) to determine the insert sequences between the ends. Plasmid and strain construction E. coli DH10B and DH1 were used for bacterial transformation and plasmid storage. A [C 2 mim]Cl-tolerant fosmid clone was used as a template to amplify E. lignolyticus DNA. Most plasmids were constructed from BglBrick vectors [29] using restriction enzymes. For plasmids containing the truncated intergenic region (pTR-9–pTR-12), the PCR product, which included the vector backbone, was phosphorylated before blunt-end self-ligation. Using circular polymerase extension cloning [30] , a 30-bp linker sequence (5′-GCTGGCTCTGCTGCAGGTTCTGGTGAATTT-3′) together with the superfolder gfp [31] was fused to the eilA 3′-end before the stop codon. eilA was expressed from low-copy plasmids (SC101), with the exception of the growth rate experiment ( Fig. 2c ), where a high-copy plasmid (ColE1) was used. An overview of primers and plasmids is given in Supplementary Tables 1 and 2 . For the production of bisabolene, plasmids were prepared according to the BglBrick cloning strategy [29] . The top portion (MevT) of the mevalonate pathway contains genes for the conversion of acetyl-CoA to mevalonate: acetoacetyl-CoA synthase from E. coli (AtoB), HMG-CoA synthase from S. cerevisiae , and an amino-terminal truncated HMG-CoA reductase from S. cerevisiae . The bottom portion (MBIS) of the mevalonate pathway contains genes for the conversion of mevalonate to FPP: mevalonate kinase from S. cerevisiae , phosphomevalonate kinase from S. cerevisiae , phosphomevalonate decarboxylase from S. cerevisiae , IPP isomerase from E. coli (idi) and farnesyl diphosphate synthase from E. coli (ispA). The codon optimized (co) (E)-γ-bisabolene synthase from Abies grandis was used [26] . Production vector pBbA5c-MevT(co)-MBIS(co)-T 1002 -P trc -Bis(co) (JBEI-6523) was constructed using JBEI-3100 (pBbA5c-MevT(co)) as a vector ( Bam HI/ Xho I) and JBEI-4174 (pBbS5k-MBIS-(co)-T 1002 -P trc -Bis(co)) as an insert ( Bgl II/ Xho I). Growth experiments E. lignolyticus or freshly transformed E. coli MG1655 (except where indicated) were grown to the stationary phase. These seed cultures were then diluted 1:200 into EZ-Rich medium (Teknova), supplemented with 1% glucose and the appropriate amounts of antibiotics (ampicillin 100 mg l −1 , chloramphenicol 12.5 mg l −1 and kanamycin 50 mg l −1 ). Cultures were grown at 37 °C in 24-well microtitre plates on the Infinite F-200 (Tecan) or Synergy 4 (BioTek) readers, or where indicated, in 200-ml baffled flasks at 200 r.p.m. Optical density was measured at a wavelength of 600 nm. The calculation of growth rates is based on the curve-fitting model of Baranyi and Roberts, which generates nearly linear growth rates in the mid-log phase [32] . Omnilog inhibitor screen Seed cultures of E. coli MG1655 containing either pTR_2 or pBbS0c as control, were diluted 1:200 into a EZ-rich medium supplemented with 12.5 mg l −1 chloramphenicol and a 1:100 dilution of redox dye A (Biolog). This stock culture was used to inoculate plates PM11 to PM20 at 100 μl per well. The plates were incubated for 22 h at 37 °C in an Omnilog plate reader. Colour changes, resulting from reduction in the redox dye, were recorded in each well. These kinetic data were analysed with OmniLog PM software (Biolog). Flow cytometry and fluorescence microscopy Stationary phase cultures expressing the EilA–GFP fusion protein were diluted 1:1,000 in PBS buffer. Using a Guava easyCyte (Millipore) flow cytometer, cells were counted (2,000 events per sample) by forward and side-scatter acquisition, and the cellular accumulation of EilA–GFP was measured by fluorescence intensity. Data acquisition was performed using InCyte software version 2.2 (Millipore). A strain of E. coli lacking GFP was used to subtract background fluorescence. For microscopy, cells were immobilized on a slide covered with a thin film of 1.5% agarose. Microscopy was performed on a Leica GM4000B fluorescence microscope. Images were taken with an Orca-HR camera (Hamamatsu) and processed with the MetaMorph 7.7 software (Molecular Devices). Bisabolene production E. coli DH1 was co-transformed with pJBEI-6523 (bisabolene pathway) and either pTR_8 ( eilAR) or pBbS0a (control) and grown to the stationary phase. As a 1:100 dilution, these strains were grown at 37 °C (200 r.p.m.) in baffled flasks containing 50 ml EZ-rich medium (1% glucose, ampicillin 100 mg l −1 and chloramphenicol 30 mg l −1 ) and the appropriate amounts of [C 2 mim]Cl to reach an optical density (OD 600nm ) of 1 for induction with 100 μM isopropylthiogalactoside (3IPTG). Three 8 ml aliquots were transferred to culture tubes and overlaid with 10% dodecane as the organic phase for bisabolene extraction. Ten microlitres of the dodecane overlays were sampled and diluted into 990 μl of ethyl acetate spiked with caryophyllene as an internal standard. The samples were analysed by GC/MS (Agilent 6,890 gas chromatography/5,973 mass spectrometry). The oven temperature was initiated at 100 °C for 0.75 min with a temperature gradient up to 250 °C at a rate of 40 °C min −1 , and held for 1 min at 250 °C. Injector and MS quadrupole detector temperatures were 230 °C and 150 °C, respectively. The MS was operated in a selected ion monitoring mode using fragment ions m/z 161, 189 and 204 for bisabolene identification and quantification. Quantification of [C 2 mim + ] by mass spectrometry E. coli harbouring an eilAR plasmid was grown to the stationary phase in M9 minimal medium containing 0.4% glucose and [C 2 mim]Cl at 0 mM, 68 mM, 136 mM or 272 mM. Media was collected before and after cultivation, centrifuged and equally diluted in 20 mM ammonium acetate and 0.2% formic acid in methanol:water (20:80 by volume) to a final [C 2 mim]Cl concentration between 5 and 50 μM. Samples (50 μl) were injected at a flow rate of 0.3 ml min −1 . Detection of [C 2 mim] + (m/z=111) was carried out using an Agilent 1,100 HPLC (Agilent Technologies Inc., Santa Clara, CA, USA) and API 2000 LC/MS/MS system (AB SCIEX, Foster city, CA, USA). Measurements were performed using a previously described method [33] with the following modifications: We used rapid direct infusion electrospray ionization mass spectrometry in the positive scan and selected ion mode. Also, our electrospray ionization conditions were 4.5-kV spray voltage with an auxiliary gas (N 2 ) flow of 20 and 8 (arbitrary units), and a heated ion transfer capillary/mass spectrometer inlet temperature of 350 °C. How to cite this article: Ruegg, T. L. et al . An auto-inducible mechanism for ionic liquid resistance in microbial biofuel production. Nat. Commun. 5:3490 doi: 10.1038/ncomms4490 (2014).